Confined propagation of covalent chemical reactions on single-walled carbon nanotubes Covalent chemistry typically occurs randomly on the graphene lattice of a carbon nanotube because electrons are delocalized over thousands of atomic sites, and rapidly destroys the electrical and optical properties of the nanotube. Here we show that the Billups–Birch reductive alkylation, a variant of the nearly century-old Birch reduction, occurs on single-walled carbon nanotubes by defect activation and propagates exclusively from sp 3 defect sites, with an estimated probability more than 1,300 times higher than otherwise random bonding to the 'π-electron sea'. This mechanism quickly leads to confinement of the reaction fronts in the tubular direction. The confinement gives rise to a series of interesting phenomena, including clustered distributions of the functional groups and a constant propagation rate of 18±6 nm per reaction cycle that allows straightforward control of the spatial pattern of functional groups on the nanometre length scale. Where and how does a molecule covalently bond to a 'π-electron sea?' This fundamental question is of central importance to the development of selective chemistries for extended carbon networks, such as single-walled carbon nanotubes (SWNTs) [1] and graphene [2] , in which π-electrons are delocalized over thousands of carbon atoms. Theoretical studies predict that the pattern of functional groups, or defects, will substantially affect the electrical and optical properties of these types of low-dimensional systems [3] , [4] . Spatially controlled chemistry may find uses in graphene edge engineering [5] , molecular lithography [6] and nanotube electrode networks [7] . Experimentally, it is challenging to control functionalization patterns in carbon nanostructures. Recent experiments have demonstrated that diazonium chemistry and oxidative reactions occur on a SWNT sidewall at completely random atomic sites [8] , [9] . The covalent modification of even a single site results in a substantial drop of electrical conductance [8] and stepwise quenching of exciton fluorescence in semiconducting nanotubes [9] . Here we show that the Billups–Birch reductive alkylcarboxylation [10] , a variant of the nearly century-old Birch reduction chemistry [11] , [12] , occurs on SWNTs exclusively, to the extent observable in our experiments, by reaction propagation from existing defects—the edge of the π-electron sea. Carbon nanotubes were homogenously dispersed in an ammonia solution of solvated electrons and covalently functionalized by alternating addition of sodium and various alkyl-halide reagents in a recycling procedure (Methods and Supplementary Fig. S1 ). The propagation mechanism of this chemistry makes it possible to progressively add new functional groups to the graphene lattice without nucleating unintended new defects. This defect-activated chemistry bears a remarkable analogy to the high reactivity of nanotube ends [13] , [14] and step edges in surface science [15] , [16] . Confinement of the reaction to carbon nanotube 'sp 3 step edges' leads to reaction fronts initiated at defect sites that ultimately propagate along the tubular direction at a constant rate ( Fig. 1a ). 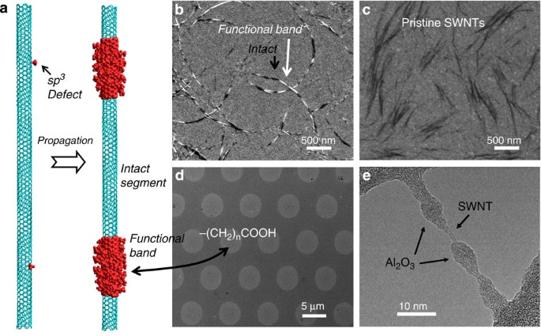Figure 1: Functional bands on SWNTs. (a) Schematic illustration of reaction propagation initiated at sp3defect centres that ultimately propagate along the tubular direction, creating sp3bands of functional groups. (b) Alkylcarboxylated nanotubes on a gold substrate imaged using a scanning electron microscope operated at 1 kV. The dark and bright contrasts closely resemble pristine nanotubes (c) and patterned carboxylic acids (d), respectively. (e) High-resolution transmission electron microscopy image of an individual SWNT-[(CH2)5COOH]ncoated with Al2O3by −COOH selective atomic layer deposition using trimethyl aluminium and H2O precursors. Figure 1: Functional bands on SWNTs. ( a ) Schematic illustration of reaction propagation initiated at sp 3 defect centres that ultimately propagate along the tubular direction, creating sp 3 bands of functional groups. ( b ) Alkylcarboxylated nanotubes on a gold substrate imaged using a scanning electron microscope operated at 1 kV. The dark and bright contrasts closely resemble pristine nanotubes ( c ) and patterned carboxylic acids ( d ), respectively. ( e ) High-resolution transmission electron microscopy image of an individual SWNT-[(CH 2 ) 5 COOH] n coated with Al 2 O 3 by −COOH selective atomic layer deposition using trimethyl aluminium and H 2 O precursors. Full size image 'Banded' SWNTs The sp 3 defect propagation mechanism was most directly illustrated by the creation of 'banded' SWNTs, with alternating segments of functionalized (sp 3 hybridized) and intact regions (which remain sp 2 hybridized) through reaction propagation that starts at defects initially present in the nanotubes or introduced during the H 2 O 2 /HCl purification process [17] . We were able to simultaneously resolve the functionalized and intact regions along the same nanotube by substrate-enhanced scanning electron microscopy (SEM) [18] . When such functionalized nanotubes were deposited on a gold substrate and imaged with a SEM electron beam of 1 kV, we observed regular alternation of bright and dark contrast along the nanotube length ( Fig. 1b ). The sharp image contrast arises from a substantial increase in the yield of secondary electrons at 1 kV because of covalent modification of the nanotube. After annealing the samples at 750 °C under flowing Ar/H 2 for 1 h, which fully recovered the pristine structure of the nanotubes, the banding structures were lost and the images show the same contrast as those of raw nanotubes ( Fig. 1c ). The brighter regions exhibit a contrast comparable to those of microcontact-printed 16-mercaptohexadecanoic acid on a gold substrate ( Fig. 1d ). On the basis of these observations, we can unambiguously attribute the bright contrast to alkylcarboxylic acid groups and the darker regions to intact nanotubes. Notably, this propagation mechanism persists even after extensive reaction. With the aid of atomic layer deposition (ALD), small segments of intact nanotubes (5–10 nm) were still frequently observed after repeating the covalent functionalization reaction 40 times. Figure 1e shows a transmission electron microscopy (TEM) image of an individual SWNT, where we selectively grew Al 2 O 3 on the carboxylic acid functional groups by alternately pulsing trimethyl aluminium and H 2 O at 150 °C. As this ALD chemistry is self-limiting and chemically selective to reactive functional groups (here carboxylic acids) [19] , [20] , [21] , the discrete Al 2 O 3 coating reflects the clustered distribution of the functional groups, −(CH 2 ) 5 COOH, along the nanotube. Propagation modes Two distinct modes of defect propagation were revealed in the length distribution of the SEM-resolved intact segments and functional bands ( Fig. 2 ). The intact segments (124±27 nm in length) follow a broad, Gaussian length distribution, suggesting a random spatial distribution of initial defects on the pristine nanotubes, as expected, at an average pitch of 212±48 nm (lower bound limit as two or more defects in proximity can develop a merged functional band). This low defect density is corroborated with negligible weight loss at elevated temperatures because of decomposition of the functional groups, low disorder peak in Raman spectra and bright fluorescence from individually dispersed pristine nanotubes. In contrast to the intact segments, the functional bands have much narrower distributions. We found that more than 80% of the 81 nanotube ends identified by SEM imaging had a functional band. These end functional bands extend 53±19 nm on average after three reaction cycles, which is approximately half the length of bands located along the nanotube sidewall (88±21 nm; Fig. 2 ). This strong length correlation arises because a defect on the nanotube sidewall will allow the propagation to occur in both directions equally, whereas there is only one possible direction to propagate from a SWNT end, the natural defect in the π-electron sea. Note that a reaction cycle in the reductive alkylcarboxylation is limited by the reductant (solvated electrons), which can be stored in the nanotube before reaction. 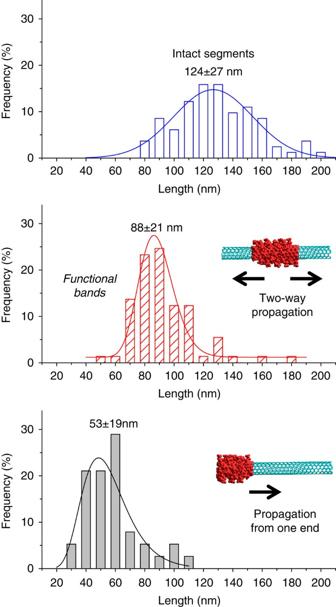Figure 2: Two modes of propagation revealed in the length distributions of intact segments and functional bands. The lengths were extracted from SEM images of the same alkylcarboxylated nanotube sample. The sample sizes are 82, 73 and 38. The curves were fitted in Gaussian, log-normal and log-normal functions with peaks at 124±27, 88±21 and 53±19 nm, respectively. The errors are standard deviations. Figure 2: Two modes of propagation revealed in the length distributions of intact segments and functional bands. The lengths were extracted from SEM images of the same alkylcarboxylated nanotube sample. The sample sizes are 82, 73 and 38. The curves were fitted in Gaussian, log-normal and log-normal functions with peaks at 124±27, 88±21 and 53±19 nm, respectively. The errors are standard deviations. Full size image Optical properties The covalently functionalized SWNTs retained some of the optical properties of pristine SWNTs ( Fig. 3 ). Optical properties of nanotubes are often completely lost because of covalent modification of the electronic band structures by even a small number of defects [9] , [22] . A defect density of ~1/10,000 (~0.001%) is sufficient to completely quench nanotube fluorescence [9] . Partial retention of the van Hove optical absorption [22] and exciton fluorescence [9] properties was made possible here even at a high degree of functionalization (~45 functional groups per 1000 carbons) because of clustered distribution of the −(CH 2 ) 5 COOH functional groups along the nanotube length, leaving intact regions of sp 2 hybridized carbons with sustained band structures ( Fig. 1a,b ). This propagation chemistry has allowed us to produce water-soluble nanotubes (up to 3,380 mg l −1 ) after 40 cycles of reaction (see Methods and Supplementary Fig. S2 ), approaching the solubility achieved only in chlorosulphonic superacid [23] . This high water solubility was previously unexpected [24] , [25] . 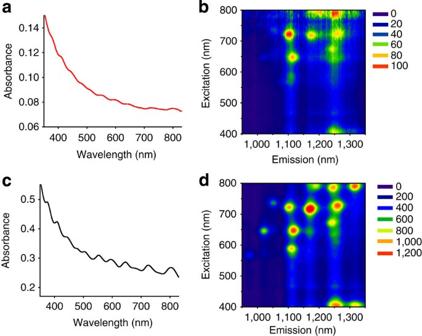Figure 3: Optical properties. (a) Visible–NIR absorption spectrum and (b) excitation-emission map of three-cycle HiPco-SWNT-[(CH2)5COOH]nin comparison with (c,d) the starting, unfunctionalized nanotubes, which were individually dispersed in D2O solutions of 1% sodium dodecylbenzenesulphonate. Figure 3: Optical properties. ( a ) Visible–NIR absorption spectrum and ( b ) excitation-emission map of three-cycle HiPco-SWNT-[(CH 2 ) 5 COOH] n in comparison with ( c , d ) the starting, unfunctionalized nanotubes, which were individually dispersed in D 2 O solutions of 1% sodium dodecylbenzenesulphonate. Full size image We propose a simple kinetic model to account for the observed propagation of functional bands ( Fig. 4 ). For free propagation from a point defect without any constraint, the number of reaction sites at the reaction front will continuously accelerate as the 'sp 3 step edge' expands. A transition occurs at a propagation length equal to the circumference of the nanotube and then at which point propagation becomes confined in a banded morphology down the length of the tube. The reaction rate becomes constant after the propagation reaches a critical length, l c ~1.5 π d, where d is the nanotube diameter—the ultimate limit of the sp 3 step edge. For a 1-nm diameter SWNT, this simple model shows that the propagation becomes confined as the reaction expands beyond ~5 nm from a defect centre. From the nanotube end functional bands, we estimate that the propagation rate is 18±6 nm per reaction cycle under the experimental conditions investigated. 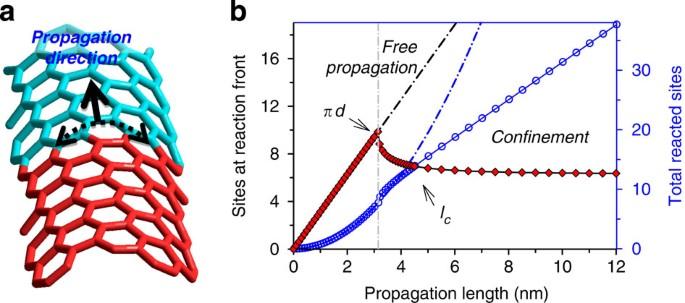Figure 4: A kinetic model of reaction propagation from a point defect on an sp2-bonded carbon lattice. (a) Schematic of the propagation front. For clarity, the functional groups are omitted. Note that for most chemistry, only a small fraction of carbon sites within the functional band are functionalized. (b) Propagation with confinement to the nanotube cylinder (solid lines) versus free propagation on an infinite sheet (dotted lines). The sites at the reaction front (red diamond) and total reacted sites (blue open circles) are computed based on geometry considerations for a 1-nm diameter nanotube. For the defect-activated reaction, the reaction rate is proportional to the number of sp3defect centres available at the reaction front, which initially increases linearly with propagation length. At a higher degree of functionalization, specifically when the propagation length reaches the circumference of the nanotubeπd, the reaction propagation becomes confined to the tubular direction. The degrees of freedom for propagation along the nanotube circumference are completely lost at a critical propagation lengthlc,~1.5πd, after which the reaction rate becomes a constant. Figure 4: A kinetic model of reaction propagation from a point defect on an sp 2 -bonded carbon lattice. ( a ) Schematic of the propagation front. For clarity, the functional groups are omitted. Note that for most chemistry, only a small fraction of carbon sites within the functional band are functionalized. ( b ) Propagation with confinement to the nanotube cylinder (solid lines) versus free propagation on an infinite sheet (dotted lines). The sites at the reaction front (red diamond) and total reacted sites (blue open circles) are computed based on geometry considerations for a 1-nm diameter nanotube. For the defect-activated reaction, the reaction rate is proportional to the number of sp 3 defect centres available at the reaction front, which initially increases linearly with propagation length. At a higher degree of functionalization, specifically when the propagation length reaches the circumference of the nanotube πd , the reaction propagation becomes confined to the tubular direction. The degrees of freedom for propagation along the nanotube circumference are completely lost at a critical propagation length l c ,~1.5 πd , after which the reaction rate becomes a constant. Full size image To more quantitatively describe this picture of reaction propagation, we calculate the relative probability of propagation with respect to the spatially random addition of new functional groups (nucleation). This parameter defines the 'purity' of reaction propagation. We can experimentally determine this parameter by estimating the lower limit number of functional groups within a functional band compared with random nucleation, if any, in the intact segments as reflected by fluorescence. For the SEM-resolved bands of a three-cycle carboxylic acid-functionalized sample ( Fig. 2 ), the corresponding average functional density, or the percentage of nanotube carbon atoms that are covalently functionalized, was ~4.5% based on the weight loss of functional groups at elevated temperatures under argon by thermogravimetric analysis (TGA). Given average lengths of 88 and 124 nm functionalized and intact regions, respectively, the functional density within the band can be calculated as at least 12%, suggesting only a fraction of the carbons within the band were functionalized. As such, an 88-nm band contains more than 1300 functional groups on average for a 1-nm diameter carbon nanotube. At this degree of functionalization, the nanotubes fluoresced with a relative quantum yield 25% that of the initial starting nanotubes ( Fig. 3 ). Because a single defect can quench the exciton fluorescence as it diffuses rapidly over 90 nm during its lifetime [9] , not more than one random nucleation on average should have occurred within the intact segments (124±27 nm). Taken together, the relative probability of propagative functionalization is at least 1,300 times higher than random nucleation. This spatial selectivity is more than 600 times higher than diazonium chemistry, the only other covalent addition chemistry whose spatial selectivity on carbon is quantified [5] . It is important to note that banding has been observed previously with scanning tunnelling microscopy on fluorinated nanotubes [26] , but the fluorination bands are densely spaced (pitch <10 nm versus the observed ~210 nm in this study), suggesting substantial contamination by random nucleation even if fluorination chemistry partially follows the propagation mechanism proposed here. To gain further insight, we repeated the reaction up to 40 cycles on CoMoCat (6,5) SWNTs and characterized the functionalized nanotubes with correlated TGA, Raman spectroscopy, Fourier transform infrared (FTIR) and water solubility measurements ( Fig. 5 ; Supplementary Figs S2-S4 ). The FTIR spectra unambiguously confirmed the rise of various infrared peaks after functionalization that are characteristic of C–H (2,800–3,000 cm −1 , C–H stretch; 1,415 cm −1 , C–H bending) and −COOH moieties (1,709 cm −1 , C=O stretch; 1,260 cm −1 , C–O stretch). The C=O stretching mode grew with increasing degrees of functionalization, in stark contrast with the featureless infrared spectrum of the pristine SWNT control ( Supplementary Fig. S3 ). Consistently, the functional density grew linearly at increasing reaction cycle, as predicted by our confined propagation model ( Fig. 5b ). 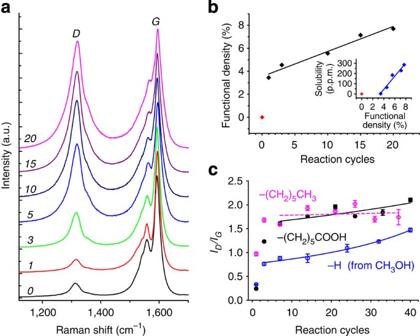Figure 5: Evolution of Billups–Birch reductive addition. Correlated (a) Raman spectra, (b) degree of functionalization as determined from weight loss in thermogravimetric analysis and water solubility (b, inset) as functions of reaction cycles for a HiPco-SWNT sample after 0–20 cycles of functionalization with Br(CH2)5COOH. The excitation line was 632.8 nm. The degree of functionalization increased as a linear function of reaction cycles. The functionalized nanotubes became water soluble at a threshold functional density of ~3.5% and thereafter increased linearly as a function of reaction cycle. (c) Effect of terminating groups on the reaction propagation probed with Raman spectroscopy. (6,5)-Enriched CoMoCat SWNTs were used for this study. The data were fitted by a rational function in the form. Figure 5: Evolution of Billups–Birch reductive addition. Correlated ( a ) Raman spectra, ( b ) degree of functionalization as determined from weight loss in thermogravimetric analysis and water solubility ( b , inset) as functions of reaction cycles for a HiPco-SWNT sample after 0–20 cycles of functionalization with Br(CH 2 ) 5 COOH. The excitation line was 632.8 nm. The degree of functionalization increased as a linear function of reaction cycles. The functionalized nanotubes became water soluble at a threshold functional density of ~3.5% and thereafter increased linearly as a function of reaction cycle. ( c ) Effect of terminating groups on the reaction propagation probed with Raman spectroscopy. (6,5)-Enriched CoMoCat SWNTs were used for this study. The data were fitted by a rational function in the form . Full size image We found that this reaction propagation mechanism is true of other functional groups as well. For all the three groups investigated, including −(CH 2 ) 5 CH 3 , −(CH 2 ) 5 COOH and −H, Raman spectroscopy revealed similar trends of reaction propagation ( Fig. 5 ), and similar banding structures were found by SEM (except −H) [18] . Covalent sidewall chemistry introduces sp 3 defect centres, which decrease the Raman oscillator strength of the tangential modes around 1,450–1,650 cm −1 (G-bands) and give rise to the so-called D-band (around 1,350 cm −1 ) [27] . This allowed us to use the D/G ratio (peak area ratio between the D-band and the G-bands) to follow the reaction progress ( Fig. 5c ). For the first three to five cycles of reaction, the D/G ratio rose exponentially, corresponding to the initial propagation from the sp 3 defect sites, which quickly convert a long nanotube into shorter segments from the Raman perspective. This is consistent with previous observations from length-sorted SWNTs that the D/G ratio rises inversely as a function of nanotube length [28] , [29] . However, as the reaction continued, the trend follows a simple form, . This trend reflects a constant growth of the number of defects ( x ), which contribute to the increase of the D-band and simultaneous decrease of the G-band intensity at relatively constant weights ( a / b ), a feature made uniquely possible by the confined propagation. What is the chemical nature of the initial defects? We do not yet have the experimental means to answer this important question, partly because the initial defect density is extremely low, ~1/10,000 (the fluorescence limit) [9] to 1/30,000 (average pitch of functional bands). However, the observed progressive alkylcarboxylation of nanotubes over at least tens of nanometres suggests that these functional groups can act as new defect centres for continued propagation of the reaction fronts. To simulate the electronic effects of a single sp 3 defect, we performed density functional theory calculations on −(CH 2 ) 5 COOH group-functionalized (5,5)-SWNT ( Fig. 6 ) and (10,0)-SWNT using periodic boundary conditions. We have used the SIESTA method [30] generalized gradient approximation of the Perdew–Burke–Ernzerhof [31] functional, a double-ζ basis set, and the standard norm-conserving Troullier–Martins pseudopotentials [32] . A Mulliken population analysis shows that the charges are localized in the carbons around the sp 3 defect and the remaining atoms have very little, almost negligible, charges ( Table 1 ; Supplementary Tables S1 and S2 ). When more electrons are added to the nanotube, as in the Birch reduction, the most significant charges are trapped around the defect site. This electronic effect extends as much as another C–C bond beyond the rings to which the functional group is attached. These results suggest that the observed propagation phenomenon originates from two effects: electrons are trapped around the defects and the trapped electrons promote localized Birch reductive addition. These are essentially the same rules that govern the regioselectivity of the Birch reduction in small aromatic compounds such as anisole [33] . In an electron-delocalized system as large as a carbon nanotube, the Birch reduction occurs by propagating the reaction fronts at the edge of the electron sea. 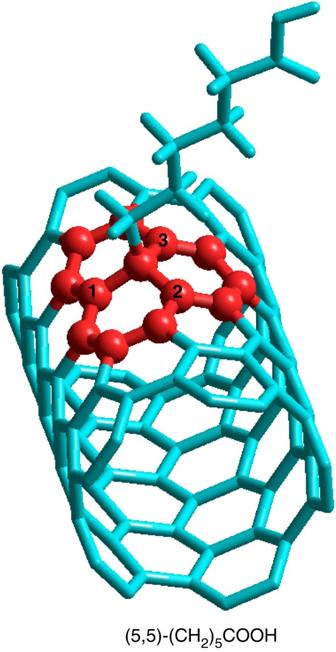Figure 6: Optimized structure of a (5,5)-SWNT with a covalently bonded −(CH2)5COOH group. The added electrons are largely localized on the highlighted carbon atoms. Figure 6: Optimized structure of a (5,5)-SWNT with a covalently bonded −(CH 2 ) 5 COOH group. The added electrons are largely localized on the highlighted carbon atoms. Full size image Table 1 Net atomic charges around a sp 3 defect site from Mulliken population analysis of a SWNT with a covalently bonded −(CH 2 ) 5 COOH group. Full size table Materials Two SWNT materials, HiPco (Rice University) and (6,5)-enriched CoMoCat (Southwest Nanotechnologies Inc.), were used in this study. HiPco-SWNTs were purified using a one-pot purification method [17] and CoMoCat SWNTs were used as received. All other reagents were purchased from Sigma-Aldrich and used without further purification. Synthesis of HiPco-[(CH 2 ) 5 COONa] n In a typical experiment, purified HiPco-SWNTs (10 mg, 0.83 mmol of carbon) were added to a flame-dried, argon-purged, 250 ml four-neck round-bottom flask fitted with a dry-ice/acetone condenser. A volume of 75 ml liquid ammonia was condensed into the flask, followed by addition of sodium (0.029 g, 1.25 mmol), which spontaneously produced a blue colour owing to solvated electrons. After stirring for 10 min, 6-bromohexanoic acid (0.975 g, 5.00 mmol) was added and the mixture was stirred overnight, while the liquid ammonia evaporated. Subsequently, 100 ml nanopure water was added to the flask and briefly sonicated. The functionalized SWNTs were collected over a 0.8-μm ATTP membrane (Millipore), redispersed in water and repeatedly extracted with hexane (20 ml) in a separatory funnel to remove salts. The hexane layer was filtered through a 0.8-μm membrane forming a buckypaper of functionalized SWNTs, which was washed with ethanol and water and dried overnight in a vacuum oven at ~80 °C. For multiple reaction cycles, the previously functionalized SWNTs were used as starting materials. Sodium and 6-bromohexanoic acid were alternately added into the flask at each reaction cycle ( Supplementary Fig. S1 ). After the first cycle, extra sodium was added to balance the loss because of the reactive −COOH groups. For each cycle, the solution was allowed to react for 1 h. Synthesis of CoMoCat-[(CH 2 ) 5 COONa] n , CoMoCat-[(CH 2 ) 5 CH 3 ] n and CoMoCat-[H] n CoMoCat SWNTs (20 mg, 1.67 mmol) were exfoliated in 75 ml liquid NH 3 by sodium (0.058 g, 2.5 mmol) and subsequently reacted with 6-bromohexanoic acid (0.650 g, 3.33 mmol), 1-iodohexane (0.706 g, 3.33 mmol) or methanol (0.533 g, 16.67 mmol). Up to 40 reaction cycles were carried out using the same procedures as described above. Three-cycle reaction and water extraction Water extraction experiments were carried out on three-cycle-functionalized HiPco-[(CH 2 ) 5 COONa] n sample, beginning with 52 mg purified HiPco-SWNTs. After functionalization, the black solid was dispersed in 80 ml basic water (pH=10.5). A volume of 10 ml hexane was then added to the dispersion and the mixture was shaken vigorously. After phase separation, the aqueous phase was collected. The hexane layer of SWNTs was filtered over 0.2 μm GTTP Isopore membrane (Millipore). This extraction process was repeated to produce 13 bottles of water-soluble SWNT solutions, the last third of which exhibited the optical properties as shown in Figure 3 . Solubility measurement The water solubility was measured by centrifugation in conjunction with ultraviolet-visible-near infrared (UV-Vis-NIR) spectroscopy. The solid samples were dispersed in basic water (pH=10) by bath sonication for 1 h. Then the aqueous solutions were centrifuged on a Beckman Coulter Microfuge 16 centrifuge (Beckman Coulter) at 1,919 g until the supernatant reached a stable, isotropic phase showing no further decrease in absorbance ( Supplementary Fig. S2 ). Spectroscopy characterization Raman scattering spectra were collected on a Horiba Jobin Yvon LabRAM HR-VIS microRaman system (Horiba) with a helium neon laser excitation source. Lower power density (~0.1 mW μm −2 ) was used to exclude laser-induced thermal effects [34] . UV–Vis–NIR spectra were measured using a PerkinElmer Lambda 1050 UV/Vis/NIR spectrophotometer (PerkinElmer). Excitation-emission maps were measured with a Horiba Jobin Yvon NanoLog spectrofluorometer (Horiba) using a liquid nitrogen-cooled InGaAs detector array. For FTIR analysis, the functionalized SWNTs were acidified with 0.5 M HCl to ensure termination with −COOH rather than −COONa. A JASCO FT/IR-4100 Spectrometer (JASCO) with an attenuated total reflectance (ATR) accessory was employed to record the FTIR spectra. Au-substrate enhanced SEM The water-soluble SWNTs were drop-cast on a gold-on-silicon substrate, air dried and then rinsed with water to remove salts. SEM was performed on a Hitachi SU-70 Schottky field emission gun scanning electron microscope (Hitachi) operating at an accelerating voltage of 1 kV, with an emission current of 34–35 μA. Atomic layer deposition Al 2 O 3 was grown on SWNT-[(CH 2 ) 5 COOH] n drop-cast on a lacey carbon copper grid (SPI) using a BENEQ TFS 500 ALD reactor. Trimethyl aluminium and deionized water were supplied as alternate 250 ms pulses from room temperature ampoules, separated by 500 ms N 2 system purges, with the reactor temperature at 150 °C. These conditions yielded a growth rate of ~1.0 Å per cycle, which was consistent with literature values [35] . Transmission electron microscopy was performed on a JEOL JEM 2100 LaB6 transmission electron microscope (JEOL) at an accelerating voltage of 200 kV. Thermogravimetric analysis TGA experiments were performed on a TA Instruments Q500 Thermogravimetric Analyzer (TA Instruments). The sample was held at 100 °C for 30 min, ramped at 10 °C min −1 to 800 °C and then held at 800 °C for 30 min under flowing Ar (100 sccm, 99.9999% purity). The functional group to carbon ratio was calculated according to the weight loss because of the thermally cleaved functional groups ( Supplementary Fig. S4 ). How to cite this article: Deng, S. et al . Confined propagation of covalent chemical reactions on single-walled carbon nanotubes. Nat. Commun. 2:382 doi: 10.1038/ncomms1384 (2011).